Multimodal label-free detection and discrimination for small molecules using a nanoporous resonator To detect chemical or biological threats, it is crucial that sensor devices can differentiate various target molecules. In general, each different sensing method has its own strengths and weaknesses due to their respective limitations. For example, although resonant sensors have high sensitivity, they are not able to discriminate target molecules. At the same time, although surface-enhanced Raman spectroscopy is a representative label-free detection method that can discriminate target molecules, its fabrication is often complex and expensive. Here we present a label-free multimodal nanoporous resonator-based system for small molecule detection and discrimination that combines the strengths of each of these sensing methods. Our approach is not only able to improve the sensitivity of the resonant sensor but it can also discriminate the target molecules. Furthermore, the fabrication process is swift (lasting <3 min) and convenient. Over the past two decades, the field of sensing has advanced to include a wide range of methods and devices for chemical, biological and environmental toxicity detection [1] . The monitoring of chemical and biological targets is important for medical diagnostics and bio-warfare applications as well as for fundamental research [2] . In addition, because of the remarkable developments that have taken place recently in the field of nanoscale research and industry, the detection range for nanotoxic materials that can adversely affect the environment and human health has been greatly increased [3] . Common method-based molecular sensing involves labelling processes such as quantum dots, fluorescent markers and dyes [4] . Although labelled detection is widely used in molecular sensing, photochemical degradation, pH-dependence, time constraints and high costs are all important considerations that can restrict the use of these methods [2] , [5] . For the various target scopes and overcoming the limitation of labelling method, current developing techniques are focused on maximizing sensitivity, label-free detection, reducing the cost and creating multimodal systems for analytical detection of target molecules [6] . Resonant sensors are highly sensitive devices that provide a method for the label-free quantitative measurement of molecular interactions [7] , [8] . The resonant sensor is one of the cantilever-based detection modes, where the binding of the molecule to the cantilever surface changes the resonant frequency of the cantilever. Thus, the resonant sensor detects the surface molecular binding directly, as the resonant frequency is a function of the cantilever mass. From this background, the resonant sensor has shown the highest potential for achieving the most sensitive measurements of molecular interactions such as enzyme–peptide interactions [9] , [10] , nucleotide interactions [11] and protein–antibody interactions [12] , [13] . Recently, we have shown that a resonant sensor was able to detect the nanotoxic material (Ag + ) in the real environment [14] . While the resonant sensing platform has high sensitivity and economic benefit due to the label-free method, the discrimination of binding molecules and time-consuming tasks for exploring in different configuration to enhance the sensitivity (using MEMS and NEMS technology) are major drawback of the resonant sensor [8] , [13] . Another well-established label-free detection method capable of single-molecule detection is surface-enhanced Raman spectroscopy (SERS). SERS is a phenomenon in which the intensity of light scattered from the molecule is amplified when light is shone on the molecules placed on nanostructured metallic surface [15] . SERS has drawn great attention as an alternative method for small molecule detection due to its multiplexing capability since the intensities and and frequencies of vibrational transitions measured in Raman spectra provide unique finger-printing spectra of molecular species [16] . Various strategies have been reported for fabricating nanostructured metallic platforms for efficient use as SERS substrates [17] , [18] , [19] . However, these nanostructured SERS substrates have several drawbacks such as a complex fabrication process, lack of uniformity at large scale and MEMS incompatibility. To overcome the above problems related to resonant sensor and SERS, we propose a novel approach for discriminating binding molecules and improving the sensitivity of resonant sensors at detection limits of 10 −9 M without amplification by making use of nanoporous sensors, in particular, multimodal nanoporous resonators (MNPR). As a result of their large surface area, nanoporous structures have been widely used for drug delivery [20] , water filtration [21] , [22] , batteries [23] and various sensor applications [24] , [25] , [26] , [27] . Herein, we adopt MNPR for small molecules detection such as p -aminothiophenol ( p -ATP) and Malachite green isothiocyanate (MG), which are representative small molecules for Raman spectroscopy to verify the SERS [28] , [29] , [30] , [31] . Moreover, the molecular weight of p -ATP (125.19 Da) is light enough to ensure the high sensitivity of MNPR by comparison with previous studies [9] , [10] , [11] . It is remarkably shown that MNPR enables one to label-free detect and discriminate small molecules, not only ~10,000 times improved sensitivity compared with commercialized resonator but also discrimination of binding molecule individually. In addition, the fabrication of MNPR is a swift (within 3 min) and convenient process that leads to reducing the cost. MNPR frabrication An MNPR for the label-free detection and discrimination of small molecules was designed by modifying a commercialized micro-resonator using an electrochemical route as shown in Fig. 1 (see Supplementary Fig. 1 ). The fabrication process for creating the MNPR involved two convenient steps. The first step was to induce Au/Ag alloy growth on a bare gold surface. Generally, the surface of a micro-cantilever is coated with a material such as gold (Au), chrome (Cr) or aluminium (Al) in order to enhance laser reflection, which will ensure a clear resonance peak and allow for high-precision atomic force microscopy (AFM) images. Au/Ag alloy was directly deposited onto the gold surface using a mixture of gold and silver-plating stock solutions over 3 min. The second step was the selective wet etching of Ag using nitric acid (HNO 3 ), which took 3 s. After gently washing process, the MNPR was ready to detect the small molecules (see Methods). These fabrication processes of the MNPR is facile to prepare comparing with other techniques. General micro/nanoporous sensors adopt the complicated procedures that include wet etching, polishing, micro/nano patterning, and so on [32] . In addition, similar de-alloying method for porous strucutre includes thermally evaporation with high vacuum system and additional enlarging the pore size process [26] . However, the fabrication process of the MNPR excludes expensive and time-consuming processes as mentioned above. Target-specific binding generally refers to antibody- or aptamer-based sensing. The binding between thiolated small molecules and a gold surface is directly detected and discriminated as means of showing proof of concept. The Au/Ag alloy deposition and the MNPR were both measured using energy-dispersive X-ray spectroscopy (EDS), see Supplementary Fig. 2 . 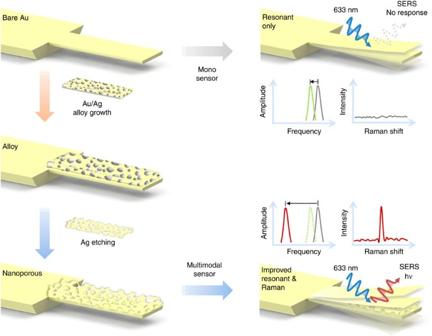Figure 1: Illustration of the fabrication procedures for the MNPR. An MNPR for the label-free detection and discrimination of small molecules was designed by modifying a commercialized micro-resonator. The modification involved two convenient steps. The first step was to induce Au/Ag alloy growth on a bare gold surface. Then, the selective wet etching of Ag using nitric acid produces a porous gold layer on the micro-resonator. Figure 1: Illustration of the fabrication procedures for the MNPR. An MNPR for the label-free detection and discrimination of small molecules was designed by modifying a commercialized micro-resonator. The modification involved two convenient steps. The first step was to induce Au/Ag alloy growth on a bare gold surface. Then, the selective wet etching of Ag using nitric acid produces a porous gold layer on the micro-resonator. Full size image Multimodal detection strategy The proposed multimodal sensing systems incorporate two detection methods. The first method is based on the shift in the resonant frequency of the cantilever upon the change of mass, which occurs when the molecule adheres to the surface. From previous studies, we have determined that the rectangular-shaped resonator exhibits resonant behaviour that is consistent with the classical elastic continuum model [14] , [33] . It is well known that mass change is a dominant factor in the resonant frequency shift of a thick micro-resonator as a result of the related molecular interactions such as molecular binding and/or molecular cleavage [9] , [14] . It means that the high sensitivity of resonance sensor is proportional to the mass increase and/or the probability of molecular adsorption. Here the sensitivity represents a general intensitiy of sensor response that is widely used for previous studies [10] , [34] , [35] . A typical mass increasing method is that of a sandwich assay that involves an attachment of a subordinate amplifier to the target molecule [36] . However, the sandwich assay is not capable of quantitatively determining the number of target molecules. In addition for small molecular sensing, investigation of adjust amplifier is difficult due to the small number of binding sites available. Thus, the increase of probability for molecular adsorption is an appropriate alternative using nanoporous structures in MNPR. It means that the MNPR has better sensitivity than the commercialized resonant sensor due to the larger surface area. The second detection method in this work is based on SERS substrates. Recently, the development of nanostructured-metal-based SERS substrates has been of great interest since the magnitude of Raman cross-section can be greatly enhanced when the Raman-active molecules are placed around a nanostructured-metal surface [37] . It is attributed to plasmonic coupling between local nanostructured-metal in close proximity, which results in huge local electromagnetic field enhancements [38] . The location of spots of giant electromagnetic field enhancement is referred to as ‘plasmonic hotspots’ [39] . Our MNPR is able to response the SERS due to lots of plasmonic hotspots and well-distributed plasmonic hotspots, which are dependent on the shape of nanostructure. Further, high-cost and complicated fabrication processes are not necessary for the MNPR manufacturing. Moreover, the target molecules were discriminated using SERS spectra, which show unique profiles for each molecule. From these standpoints for high sensitivity and target molecule discrimination, though bare resonator was able to detect the small molecules ( p -ATP) using a resonant frequency shift only, the bare resonator showed a deficiency for both points. In contrast, nanoporous structure of MNPR led to an improved resonant frequency shift and response of SERS. Further, the MNPR solves the shortcoming of each technique. In the viewpoint of the resonant sensor, unrecognized bound molecules are the critical drawback. Furthermore, SERS also have the drawback in which the sensitivity is dependent on the shape of the nanostructure. Consequently, our sensing platform complements to each technique using discrimination of target molecules and enhancement of sensitivity. MNPR optimization In order to find the optimal conditions for small-molecule detection, the surface morphologies and Raman-mapped images of MNPRs were obtained using tapping-mode AFM (tmAFM) and confocal Raman microscopy on the Au-containing plating stock solutions, respectively. 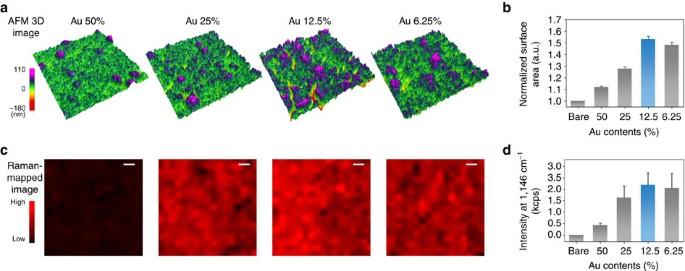Figure 2: Optimization of MNPR. (a) Tapping-mode 3D AFM image of MNPRs with respect to the Au content of the plating stock solution. The size of all images was 3 × 3 μm. (b) Normalized surface area with respect to the Au contents. For the statistical data, normalized surface areas of 10 different MNPRs were measured for each percentage. Each error bar indicates the s.d. Blue bar indicates the normalized surface area of a MNPR with optimal Au content (12.5%). (c) Confocal Raman mapped images of MNPRs with respect to the Au content after deposition of 10−4M ofp-ATP molecules (scale bar 1 μm). The Raman signal was imaged between 1,140 and 1,145 cm−1. (d) SERS intensity with respect to the Au contents usingp-ATP molecules at 1,146 cm−1. For the statistical data, intensities at 1,146 cm−1of 10 different MNPRs were measured for each percentage. Each error bar indicates the s.d. Blue bar indicates the SERS intensity of a MNPR with optimal Au content (12.5%). Figure 2a showing the surface morphologies of MNPRs in the three-dimensional (3D) images are rendered in red, green and violet colours, which indicate the deep (approximately −180 nm), flat (0 nm) and towering (~110 nm) areas, respectively. As mentioned above, in the point of view for resonant sensor, high sensitivity is proportional to a large surface area since a larger surface area corresponds to an increase in the molecular adsorption probability. From the tmAFM 3D images, it is noticed that the decreased content of Au led to an increase in the surface area until the solution reached 12.5% (1/8) of Au/Ag plating stock solution because vacancy among gold foams is increased. The surface area of lowest Au content (6.25%) was only slightly decreased because the number of vacancies was sufficiently large to produce what could be considered a dead volume. In order to compare the surface areas definitively we employed a normalized surface area for Au content ( Fig. 2b ). The size of all tmAFM 3D images was 3 × 3 μm, which was the standard area for normalization. Here the normalized surface area was described as A n = A m / A b , where A m and A b are the surface area of MNPR and bare resonator, respectively. As shown the Fig. 2b , the optimal Au content is 12.5% in stock solution, which gave a normalized surface area of 1.532±0.242 (blue bar, A n ±s.d.). To increase the statistical validity, normalized surface area of 10 different MNPRs were measured for each Au content. In parallel to the surface area analysis of MNPRs using AFM analysis, estimation of electrochemically active surface area was additionally investigated using cyclic voltammetric analysis of gold oxide formation and stripping ( Supplementary Fig. 3 ). Significant anodic current takes place at a potential above ~1.7 V due to surface oxide formation. Thereafter, the electric charge transferred during the reduction of gold oxide (reduction peak ~0.7 V) was used to estimate the electrochemically active surface area. From these results, 12.5% of Au content was chosen for use in the MNPR fabrication. Even though the normalized surface area is not able to present an absolute value for MNPR from the tmAFM imaging method, the tendency of the surface area was able to be observed using tmAFM analysis. In order to determine the optimal conditions for SERS response, confocal Raman-mapped images were also observed with respect to Au content, which were widely used for evaluation of the SERS enhancement uniformity ( Fig. 2c ) [40] . In order to evaluate the enhancement of the Raman scattering intensity for each sample, p -ATP (100 μM) was deposited on each sample and the intensity of the Raman signal between 1,140 and 1,145 cm −1 that was mapped. It is noticable that the peak c.a. 1,142 cm −1 existed with considerable enhancement by –N=N– stratching mode (so called ‘b 2 mode’) of 4,4′-dimercaptoazobenzene (DMAB), which was oxidatevly transformed from p -ATP during SERS measurement [28] , [41] , [42] . Raman-mapped images of MNPRs display that the Raman signal of highest Au content (50%) show relatively weaker signal enhancement than samples with lower Au content due to the lack of plasmonic hotspots. Moreover, although the nanostructure of MNPRs was randomly organized, the enhancement of the Raman scattering was almost evenly distributed because the diameter of the illuminating laser beam (1 μm) was sufficiently large to equalize the local structures. Figure 2d shows the peak intensities of SERS from each MNPR. Further, for the statistical validity we measured the intensities at 1,146 cm −1 of 10 different MNPRs of each Au percentage. The optimal Au content utilized for the MNPRs as SERS substrates is 12.5% of Au content as seen from the confocal Raman-mapped images. Figure 2: Optimization of MNPR. ( a ) Tapping-mode 3D AFM image of MNPRs with respect to the Au content of the plating stock solution. The size of all images was 3 × 3 μm. ( b ) Normalized surface area with respect to the Au contents. For the statistical data, normalized surface areas of 10 different MNPRs were measured for each percentage. Each error bar indicates the s.d. Blue bar indicates the normalized surface area of a MNPR with optimal Au content (12.5%). ( c ) Confocal Raman mapped images of MNPRs with respect to the Au content after deposition of 10 −4 M of p -ATP molecules (scale bar 1 μm). The Raman signal was imaged between 1,140 and 1,145 cm −1 . ( d ) SERS intensity with respect to the Au contents using p -ATP molecules at 1,146 cm −1 . For the statistical data, intensities at 1,146 cm −1 of 10 different MNPRs were measured for each percentage. Each error bar indicates the s.d. Blue bar indicates the SERS intensity of a MNPR with optimal Au content (12.5%). Full size image MNPR characterization In order to investigate the characteristic properties of the MNPRs, scanning electron microscopy (SEM), tmAFM and Raman spectroscopy are used to determine their morphological properties, resonance behaviour and SERS responses ( Fig. 3 ). 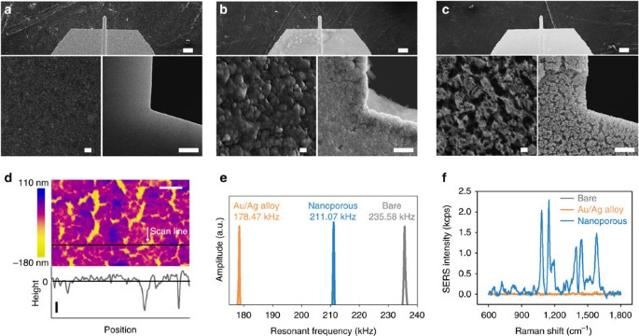Figure 3: Characterization of MNPR. SEM image of each resonator surface: (a) bare Au surface, (b) Au and Ag alloy surface, and (c) nanoporous surface (in each panel, top scale bar is 100 μm, bottom right scale bar is 1 μm and bottom left scale bar is 100 nm). (d) tmAFM image of nanoporous surface and its corresponding height profile (horizontal scale bar is 500 nm and vertical scale bar is 500 nm). (e) Resonant frequency of bare Au, Au/Ag alloy, and nanoporous state of resonator. (f) SERS response of bare Au, Au/Ag alloy, and nanoporous state of resonator using 10−4M ofp-ATP molecules. Figure 3a–c shows SEM images of the bare Au surface, the Au/Ag alloy deposition surface and the MNPR surface, respectively. The scale bars of top, right and left indicate 100 μm, 1 μm and 100 nm, respectively. Flat surface morphology was observed in the commercialized resonator ( Fig. 3a ). After the Au/Ag alloy deposition was complete, the surface roughness was seen to have increased relative to the bare Au surface ( Fig. 3b ). Here the ratio of Au content in Au and Ag plating stock solutions was 12.5%, which was optimal for small molecule sensing as previously discussed. Ultimately, the nanoporous Au substrate was observed after the Ag-etching step was performed using nitric acid ( Fig. 3c ). The nanoporous structures were described as physically having two parts: deep trenches and small holes, which were the space for dissolved Ag. The width of deep trenches and small holes were 100–500 nm and <100 nm, respectively. For the depth measurement, we have employed the tmAFM images and profile for the MNPR surface ( Fig. 3d ). From the height profile, the average depth of the deep trenches and small holes was ~135 nm and ~30 nm, respectively (>20 profiles measurements). Herein, height profiles were only able to show the trend for the depth due to the limitation imposed by the radius of the tip of the micro-cantilever. The resonance behaviours of the bare Au state (grey line), Au/Ag alloy deposition state (orange line) and MNPR (blue line) are shown in Fig. 3e . All these resonance peaks were determined using the same commercial cantilever using the fabrication protocol. It is shown that a decrease in the resonance frequency indicates an increase of mass relative to the bare Au surface, which is due to the Au/Ag alloy deposition [33] . In contrast, the resonance peak increases as a result of the Ag etching, which is indicative of the related mass decrease. However, the resonance peak of the MNPR was still lower than that of the bare cantilever because of the Au nanoporous structures that remained. The final characteristic property of the MNPR measured was the SERS response of each state after deposition of p -ATP molecules (100 μM) ( Fig. 3f ). For the case of the bare Au state or the Au/Ag alloy deposition state, the Raman spectrum is not observed because the quantity of the absorbed p -ATP on the sample substrate is too small to be observed using normal Raman scattering techniques. However, in case of the MNPR, the Raman spectrum is observed due to the enhancement of the Raman scattering. Figure 3: Characterization of MNPR. SEM image of each resonator surface: ( a ) bare Au surface, ( b ) Au and Ag alloy surface, and ( c ) nanoporous surface (in each panel, top scale bar is 100 μm, bottom right scale bar is 1 μm and bottom left scale bar is 100 nm). ( d ) tmAFM image of nanoporous surface and its corresponding height profile (horizontal scale bar is 500 nm and vertical scale bar is 500 nm). ( e ) Resonant frequency of bare Au, Au/Ag alloy, and nanoporous state of resonator. ( f ) SERS response of bare Au, Au/Ag alloy, and nanoporous state of resonator using 10 −4 M of p -ATP molecules. Full size image Resonant sensing To investigate the small-molecule capturing capability of the MNPR, we prepared different p -ATP concentrations for use in quantitative analysis ( Fig. 4 ). In this experiment, we compared the normalized resonant frequency shift between a commercial resonator (grey bar) and MNPR (blue bar) with respect to p -ATP concentrations from 10 μM to 1 nM. First, in order to characterize the capturing sensitivity, we normalized the resonant frequency of the MNPR due to the diverse initial resonance of each individual cantilever. The normalized resonant frequency is described as ω m =( ω c − ω n )/ ω b × 100, where ω c and ω n are the resonant frequencies of the capturing of a small molecule using MNPR and the Au nanoporous state, respectively, and ω b is the resonant frequency of the bare Au state resonator. In Fig. 4 , the normalized resonant frequency shift of the MNPR shows high sensitivity to the p -ATP compared with the bare Au resonator using well-known gold–sulphur chemistry. Here the limit of detection (LOD) of MNPR is 1 nM (0.110±0.091, ω m ±s.d. ), which shows a ~10,000 times improvement over the LOD of the commercial resonator (10 μM, 0.167±0.03). As the molecular weight of p -ATP (MW=125.19 Da) is extremely small, the normal resonator is not able to track the concentration ( Supplementary Fig. 4 ). For the statistical validity and reproducibility of preparation process, resonant frequencies of five different MNPRs were measured for each concentration [14] , [43] . The 0 M measurement indicates the control experiment using only ethanol solution (0 M, 0.010±0.023 for MNPR and 0.008±0.021 for the commercial resonator, Supplementary Fig. 5 ). The proposed sensing platform has better sensitivity than our previous studies, which used a commercial method that was only able to amplify the mass [9] , [10] , [14] . Moreover, our MNPR has a possibility for increasing the sensitivity using a properly designed mass amplifier [14] , [43] . In this experiment, the detection limit of p -ATP increase to 10 pM using sandwich assay amplifier ( Supplementary Fig. 6 ). Here, the PEG (5 kDa) molecules acted as a mass [9] . 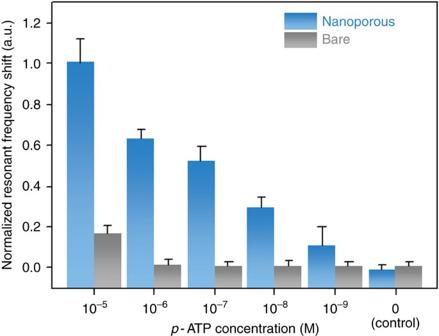Figure 4: Resonant sensing using MNPR. Normalized resonant frequency shift of MNPR and bare resonator with respect top-ATP concentration. The blue bars and grey bars indicate the normalized resonant frequency shift of MNPR and bare resonator, respectively. 0 M indicates the control experiment. For the statistical data, resonant frequencies of five different MNPR were measured for each concentration. Each error bar indicates the s.d. Figure 4: Resonant sensing using MNPR. Normalized resonant frequency shift of MNPR and bare resonator with respect to p -ATP concentration. The blue bars and grey bars indicate the normalized resonant frequency shift of MNPR and bare resonator, respectively. 0 M indicates the control experiment. For the statistical data, resonant frequencies of five different MNPR were measured for each concentration. Each error bar indicates the s.d. Full size image SERS sensing In the viewpoint of a resonator, though MNPR have a magnificent sensitivity, MNPR shows constraints such as target-molecule discrimination due to the characteristic of resonance-based sensing method. However, MNPR does allow for another method of discrimination target molecules. For the proof of concept, we have taken into account the SERS response using MNPR because Raman scattering gives molecule-specific information ( Fig. 5 ) [16] . Prior to the discrimination of captured small molecules using MNPR, we investigated the feasibility of utilizing MNPR as a SERS substrate using confocal Raman mapping on MNPR after small-molecule capture ( p -ATP, 100 μM) ( Fig. 5a ). We mapped the intensity of the SERS signal from a 10 × 10 μm square at the centre-neck site of the resonator. It was shown that the significant SERS signal was fairly uniformly observed in comparison with several reports (note the brightness of the red colour at bottom image) [17] , [40] . Therefore, we measured the SERS signal of the MNPR after the capture of two different small molecules for various solution concentrations: p -ATP and MG ( Fig. 5b ). The upper graph in Fig. 5b is the SERS signal of MNPR after the capture of p -ATP. The characteristic Raman scattering peak at 1,079 cm −1 (a 1 band of p -ATP) and three additional peaks at 1,145, 1,383 and 1,436 cm −1 (b 2 band of DMAB, oxidatively transformed from p -ATP) were observed [28] , [41] , [42] . In contrast, after the capture of MG, the characteristic Raman scattering peaks at 1,180, 1,370 and 1,618 cm −1 were observed [44] . The characteristic Raman scattering peaks of the two captured small molecules are different. Furthermore, we expect that molecular-specific discrimination of any captured small molecule is possible using the SERS measurement of the MNPR. We also depicted peak SERS intensity of each molecule with different concentrations for quantitative analysis ( Fig. 5c,d ). The LOD for SERS discrimination of p -ATP ( Fig. 5c ) is 1 μM and for MG ( Fig. 5d ) the LOD is 100 nM. The LOD of MG is 10-fold greater than that of p -ATP because the electronic transition of MG is in resonance with the frequency of the incident laser light [45] . 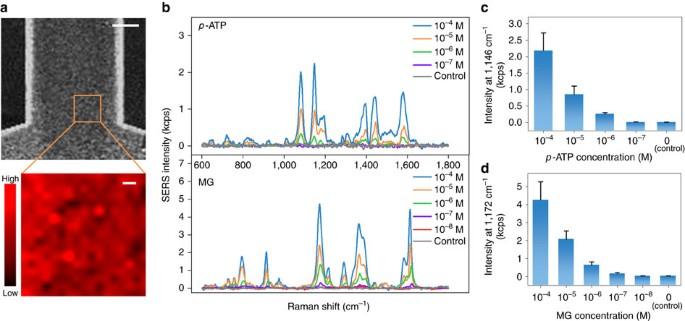Figure 5: SERS sensing using MNPR. (a) SEM and confocal Raman-mapped image of MNPR usingp-ATP molecules. Raman signal was imaged between 1,140 and 1,145 cm−1(top scale bar is 10 μm and bottom scale bar is 1 μm). (b) SERS spectra of MNPR with different concentrations ofp-ATP and MG. (c) SERS intensity (1,146 cm−1) of MNPR against p-ATP concentration. For the statistical data, five different MNPR were measured for each concentration. Each error bar indicates the s.d. (d) SERS intensity (1,172 cm−1) of MNPR against MG concentration. The laser (λ=633 nm) on the MNPR was 500 μW and the integration time was 10 s. For the statistical data, five different MNPR were measured for each concentration. Each error bar indicates the s.d. Figure 5: SERS sensing using MNPR. ( a ) SEM and confocal Raman-mapped image of MNPR using p -ATP molecules. Raman signal was imaged between 1,140 and 1,145 cm −1 (top scale bar is 10 μm and bottom scale bar is 1 μm). ( b ) SERS spectra of MNPR with different concentrations of p -ATP and MG. ( c ) SERS intensity (1,146 cm −1 ) of MNPR against p-ATP concentration. For the statistical data, five different MNPR were measured for each concentration. Each error bar indicates the s.d. ( d ) SERS intensity (1,172 cm −1 ) of MNPR against MG concentration. The laser ( λ =633 nm) on the MNPR was 500 μW and the integration time was 10 s. For the statistical data, five different MNPR were measured for each concentration. Each error bar indicates the s.d. Full size image In summary, we have reported a novel approach based on MNPR that has not only shown high sensitivity but also excellent target molecule discrimination. The optimal fabrication process of MNPR was determined by carrying out a surface area analysis using Raman mapped images provided by tmAFM and confocal Raman microscopy. The LOD of MNPR is 1 nM of which sensitivity is 10,000 times higher than commercial resonator to small-molecule detection. It was also shown that MNPR was able to discriminate the binding molecules 1 μM for p -ATP and 100 nM MG molecules using SERS response. It is noted that until recently these methods have not been available, which can provide multimodal high-sensitive detection and discriminational information of binding molecules. It is due to the limitation of conventional detection methods. However, as described in this work, MNPR is able to endow an insight into fusion detection method, which accumulates the advantages of label-free sensing methods from merely simple and swift fabrication process. Furthermore, because of AFM–Raman technique [46] the MNPR has possibility for commercializing toward various target molecules. In the long run, it is implied that MNPR may enable not only basic label-free sensitive sensor platform capable of revealing an insight into the efficacy of general biological, chemical, environmental and blood sensor [47] , [48] but also the fiducial point for multimodal detection. MNPR fabrication For the fabrication of MNPR, Au/Ag alloy was electrochemically deposited on the Au surface of micro a cantilever and Ag was selectively etched into the surface. The PPP-NCHAu (NANOSENSORS, Switzerland) cantilever was used as a resonator with dimensions of 30 × 4 × 125 μm 3 (width × thickness × length) and a force constant of ~42 N m −1 . A metallic layer of (Au) was coated on both sides of the resonator that improved the contact area. The resonant frequency of the resonator was ~240 kHz, which was an appropriate frequency for cantilever sensors in air [9] , [14] . However, for quantitative analysis we normalized the resonant frequency of the resonator due to different initial values of the various cantilevers [14] . Prior to electrochemical deposition, the Au-coated micro resonators were sequentially cleaned with acetone, ethanol and deionized water. In order to determine the exposed area for Au/Ag alloy deposition, the non-exposed area was passivated using lacquer. Electrochemical experiments were performed using a potentiostat (CompactStat, Ivium) that was controlled by a computer. A conventional three-electrode system was used for this experiment with a platinum (Pt) wire counter electrode, an Ag/AgCl (1 M KCl) reference electrode and a working electrode. Au/Ag alloy was electrochemically deposited by using a mixture of gold and silver-plating stock solutions. A gold-plating stock solution was prepared by dissolving 20 mM gold cyanide in an aqueous media and the pH was controlled using Na 2 CO 3 and the silver-plating stock solution was prepared by dissolving 20 mM silver cyanide rather than gold cyanide. A mixture of gold-plating stock solution and silver-plating stock solution was prepared in various ratios (Au 50, 25, 12.5 and 6.25%). The Au/Ag alloy was deposited in a mixture solution at −0.8 V versus Ag/AgCl for 180 s. The reaction was performed in a temperature-controlled vessel at 10 °C. Thereafter, selective etching of Ag was performed by immersion of as-prepared Au/Ag alloy-deposited micro-cantilever in nitric acid (HNO 3 ) for 2 s. After selective etching, the MNPR was washed with ethanol and triple-distilled water (Millipore, Bedford, MA, pH 7.5) several times until it was clean. After the washing process was complete, the MNPR was dried under vacuum for 6 h at room temperature. Synthesis of PEG conjugated p -ATP Synthesis of PEG-conjugated p -ATP was carried out by well-known amine–NHS carboxylate-based method. In detail, p -ATP and monomethoxy-NHS-activated PEG (mPEG-NHS; MW: 5k) were allowed to react in chloroform for 24 h at room temperature. Then, the resultatnt products were dialysed (MWCO: 1k) to exlude unreacted p -ATP ( Supplementary Fig. 6 ). TmAFM and SEM images and analysis TmAFM measurements were performed using an Innova (Bruker Corp., CA, USA) with a NanoDrive controller (Bruker Corp) in air at ambient temperature and pressure. The clear images were obtained using a closed-loop scanner, which allows precise, reproducible images of each state. For an accurate imaging, the ultra-sharp tip which name is SSS-NCHR (NANOSENSORS, Switzerland) cantilever tip was used for recording the two-dimensional (2D) and 3D images. The tip radius of this cantilever was ~2 nm and the resonant frequency was ~300 kHz. All images were 3 × 3 μm in size with a scanning frequency of at 0.8 Hz. Two-dimensional levelling processes were performed for all images using SPM Lab Analysis software V 7.00 (Bruker Corp.). The surface area analysis was performed using Nanoscope analysis software V 1.20 (Bruker Corp.). The morphology of the MNPRs was observed by FE-SEM (JSM-6500F, JEOL). p -ATP detection comparison and control experiment For the resonant frequency shift of both MNPR and the bare resonator due to the p -ATP (Sigma-Aldrich Chemicals) absorption, AFM was used to measure (Innova with Nanodrive controller). The p -ATP had an amine group (NH 2 ) and thiol group (SH) on both ends. In order to facilitate p -ATP adsorption on the MNPR and the bare resonator surface, both resonators were immersed in the ethanol-based p-ATP buffer solution for 1 h. The p -ATP molecules were attached on both the Au surface (bare resonator and the MNPR) using well-known gold–sulpgur chemistry. In order to confirm the possibility of physical absorption on the surface, we prepared ethanol solution without p -ATP ( Supplementary Fig. 5 ). We observed that the resonant frequency shifts of the bare resonator and the MNPR did not occur in the control experiment ( Fig. 4 , 0 M). This resonant frequency shift shows the reliability results comparing with our previous work [9] , [14] , [43] . The statistical data were normalized for the resonant frequency shift of five different resonators and data were obtained at each concentration. Raman spectra imaging and analysis Raman spectroscopy measurements were performed using confocal Raman microscopy (LabRAM ARAMIS, Horiba). A × 100 microscope objective (Nikon, NA=0.95) and a He-Ne laser ( λ =633 nm) were used to obtain the high-quality images. The laser power on the sample was ~50 μW, and the integration time was 10 s. A silicon wafer with a Raman band at 520 cm −1 was used to calibrate the spectrometer. For confocal Raman imaging spectroscopy, the laser power on the sample was ~0.5 mW, the integration time was 1 s per spectrum and the scanning step was 0.5 μm. LabSpec 5 software (Horiba) was used for spectral and image processing and analysis. EDS measurement FE-SEM and EDS were performed with a FE-SEM (JSM-7100F, JEOL) equipped with an energy-dispersive X-ray analyser at an accelerating voltage of 20 kV ( Supplementary Fig. 2 ). Electrochemical estimation of surface area Electrochemical experiments for estimation of surface area were also performed using a potentiostat (CompactStat, Ivium). A conventional three-electrode system was used for this experiment with a platinum (Pt) wire counter electrode, an Ag/AgCl (1 M KCl) reference electrode and a working electrode (Bare, Au 50%, Au 25%, Au 12.5% and Au 6.25%). Cyclic voltammetry was used to estimate the electrochemically active surface area. Cyclic voltammetries were performed in 0.5 M sulphuric acid in the potential range between −0.2 V (initial value) and 1.8 V (versus Ag/AgCl) at a scan rate of 10 mV s −1 . For each working electrode, 20 cycles were performed in order to achieve reliable measurements. For surface-area esimation, gold oxide reduction peak (0.6 to 1.2 V) was integrated. How to cite this article: Park, J. et al. Multimodal label-free detection and discrimination for small molecules using a nanoporous resonator. Nat. Commun. 5:3456 doi: 10.1038/ncomms4456 (2014).